Sirt1 improves healthy ageing and protects from metabolic syndrome-associated cancer Genetic overexpression of protein deacetylase Sir2 increases longevity in a variety of lower organisms, and this has prompted interest in the effects of its closest mammalian homologue, Sirt1, on ageing and cancer. We have generated transgenic mice moderately overexpressing Sirt1 under its own regulatory elements (Sirt1-tg). Old Sirt1-tg mice present lower levels of DNA damage, decreased expression of the ageing-associated gene p16 Ink4a , a better general health and fewer spontaneous carcinomas and sarcomas. These effects, however, were not sufficiently potent to affect longevity. To further extend these observations, we developed a metabolic syndrome-associated liver cancer model in which wild-type mice develop multiple carcinomas. Sirt1-tg mice show a reduced susceptibility to liver cancer and exhibit improved hepatic protection from both DNA damage and metabolic damage. Together, these results provide direct proof of the anti-ageing activity of Sirt1 in mammals and of its tumour suppression activity in ageing- and metabolic syndrome-associated cancer. Overexpression of protein deacetylase Sir2 in yeasts, flies and worms has the remarkable effect of extending longevity [1] , [2] . Mammals have evolved a family of Sir2-related proteins known as sirtuins and composed of seven members (Sirt1-7), of which Sirt1 is the closest homologue to Sir2 [2] . However, little is known at present about the impact of mammalian Sirt1 on ageing [3] . Regarding cancer, available genetic evidence supports a tumour-suppressor role of Sirt1 [4] . In particular, decreased Sirt1 activity accelerated the tumour-prone phenotype of p53-heterozygous mice [5] and, reciprocally, overexpression of Sirt1 in lymphocytes delayed the development of radiation-induced lymphomas in p53-heterozygous mice [6] . Moreover, Sirt1 binds and deacetylates β-catenin, thus cancelling its oncogenic transcriptional activity and decreasing intestinal tumour development [7] . Although the above results are of obvious importance, the impact of systemic Sirt1 upregulation on ageing and on ageing-associated cancer remains to be determined. This is particularly relevant given the ongoing efforts to develop drugs that stimulate Sirt1 activity, including resveratrol and SRT1720 [8] , [9] , [10] . Regarding these latter compounds, it is controversial whether they activate Sirt1 directly [8] , [9] , [11] , [12] . Alternatively, resveratrol may upregulate Sirt1 through indirect mechanisms that could involve AMPK [13] , [14] . It has been previously reported by others and us that transgenic mice systemically overexpressing Sirt1 ( ∼ 3-fold) are protected from the physiological damage produced by a high-fat diet (HFD) [15] , [16] . These observations are further reinforced by the phenotype of mice deficient in Dbc1, a negative regulator of Sirt1, which also shows systemic activation of Sirt1 and protection from HFD-induced damage [17] . At a molecular level, protection against HFD has been reported to reflect the activity of Sirt1 as a negative regulator of nuclear factor-κB (NF-κB) [15] , [17] and as a positive effector of PGC1α [15] and FoxO1 [16] . Chronic exposure to high levels of dietary fat results in a multi-systemic deterioration known as metabolic syndrome, which is characterized by insulin resistance, liver steatosis, atherogenic cardiovascular disease, dyslipidaemia and systemic inflammation, which may lead to fatal diseases such as liver cancer and heart failure [18] , [19] . Given the prevalence of metabolic syndrome in the adult and aged human population [20] , it is of interest to determine the impact of Sirt1 upregulation on metabolic syndrome-associated cancer. In this study, we examine the ageing and longevity of Sirt1-tg mice, as well as their susceptibility to spontaneous cancer and to liver cancer associated with metabolic syndrome. Our results indicate that Sirt1 exerts antiageing activity in mammals, although this effect is not sufficiently potent to extend longevity, at least at the levels of overexpression achieved in our mice. Sirt1-tg mice are protected from the development of ageing-associated diseases such as glucose intolerance, osteoporosis and cancer. Moreover, Sirt1 provides a strong protection against liver cancer development in the context of metabolic syndrome. Normal longevity and decreased spontaneous cancer To evaluate the impact of Sirt1 on mammalian ageing, we analysed two independent lines of Sirt1 transgenic mice carrying different, but overlapping genomic DNA segments ( Supplementary Fig. S1a ). These two lines, named here as Sirt1-tgA [15] and Sirt1-tgB, overexpress ∼ 3-fold Sirt1 mRNA across all tissues tested ( Supplementary Fig. S1b) , and present detectably higher levels of Sirt1 protein ( Supplementary Fig. S2a–c ), as well as an increase in hepatic Sirt1 activity measured by the lower levels of acetylated lysine 310 of p65RelA ( Supplementary Fig. S2c ), a known target of Sirt1 deacetylase activity [21] . In agreement with their similar levels of Sirt1 upregulation, both transgenic lines displayed similar phenotypes regarding protection from HFD, such as, decreased adipose tissue inflammation ( Supplementary Fig. S3a) , improved glucose tolerance ( Supplementary Fig. S3b and ref. [15] ), and protection from hepatic steatosis ( Supplementary Fig. S3c and ref. [15] ), as well as increased sensitivity to lipopolysaccharide shock under standard diet ( Supplementary Fig. S4 and ref. [15] ). To determine the impact of Sirt1 upregulation on longevity, we followed up cohorts of the two lines, together with their corresponding wild-type (WT) controls. All cohorts had the same uniform but hybrid genetic background (C57BL6/CBA 87.5:12.5%). The corresponding survival curves are represented by either separating the two lines or pooling them together. Pooling allowed us to achieve a cohort size per genotype and sex of n >40, which provides sufficient statistical power to reliably detect differences greater than 10% in mean lifespan [22] . The survival curves of Sirt1-tg(A+B) and WT(A+B) were indistinguishable for both male and female mice ( Fig. 1a ). When male and female mice were grouped together, the number of WT mice and tg mice was n >100 and, again, no differences were detected in survival ( Fig. 1a ). Moreover, no significant differences were found between Sirt1-tg mice and their corresponding WT controls when each line was analyzed separately ( Fig. 1a ). We conclude that systemic threefold upregulation of Sirt1 has no detectable impact, neither detrimental nor beneficial, on mouse longevity. 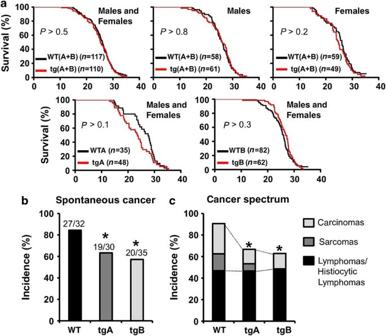Figure 1: Normal lifespan but enhanced cancer protection in Sirt1-tg mice. (a) Survival of cohorts of mice of the indicated genotypes. Log-rank tests indicated that Sirt1-tg mice were not statistically different from WT mice (P>0.05). (b) Spontaneous cancer incidence. Statistical significance versus WT mice was calculated using Fisher's exact test: *P<0.05. (c) Cancer spectrum. Statistical analysis refers to the combined incidence of carcinomas and sarcomas versus WT mice using Fisher's exact test: *P<0.05. Figure 1: Normal lifespan but enhanced cancer protection in Sirt1-tg mice. ( a ) Survival of cohorts of mice of the indicated genotypes. Log-rank tests indicated that Sirt1-tg mice were not statistically different from WT mice ( P >0.05). ( b ) Spontaneous cancer incidence. Statistical significance versus WT mice was calculated using Fisher's exact test: * P <0.05. ( c ) Cancer spectrum. Statistical analysis refers to the combined incidence of carcinomas and sarcomas versus WT mice using Fisher's exact test: * P <0.05. Full size image Detailed histopathological analyses of old moribund mice revealed a lower incidence of malignant tumours in Sirt1-tg mice, compared with WT mice of both lines ( Fig. 1b ). Remarkably, the suppressive effect of Sirt1 on malignant tumours was restricted to carcinomas and sarcomas (mostly osteosarcomas), whereas it had no effect on the incidence of lymphomas and histiocytic lymphomas (the latter also known as histiocytic sarcomas) ( Fig. 1c ). It is important to mention that most spontaneous carcinomas and sarcomas were in general of small size (as was the case of liver or lung carcinomas) or affected non-vital organs (such as Harderian gland carcinomas in the eyes or osteosarcomas in the limbs). Therefore, despite their malignancy, most carcinomas and sarcomas were at a stage of dissemination that is unlikely to be the primary cause of death. This is in contrast to spontaneous lymphomas, which had similar incidences in WT and tg mice, and were highly aggressive and the likely cause of death. In summary, these results indicate that Sirt1 upregulation provides protection from spontaneous carcinomas and sarcomas, but not from spontaneous lymphomas. Conceivably, the lack of effect of Sirt1 on spontaneous lymphomas could mask a putative effect of Sirt1 on longevity. Improved healthy ageing To examine the impact of Sirt1 on ageing, we began by examining a physiological parameter related to metabolic syndrome, namely, ageing-associated glucose intolerance [23] . Young (3 months old) WT and Sirt1-tg mice under a standard diet showed similar performance in glucose-tolerance tests [15] , [16] (see also Supplementary Fig. S3b ). Interestingly, at 1.5 years of age, WT mice already showed evidence of glucose intolerance, whereas transgenic Sirt1 mice preserved a significantly better glucose uptake ( Fig. 2a ). These results indicate that Sirt1 confers protection against ageing-associated metabolic damage under standard diet and, together with previous data on mice under an HFD [15] , [16] , [17] , reinforce and extend the concept that Sirt1 is a general protector against metabolic damage. 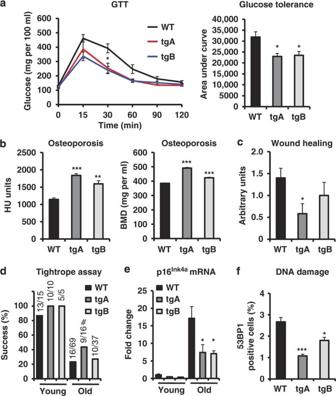Figure 2: Improved healthy ageing in Sirt1-tg mice. (a) Glucose tolerance test (GTT) in 1.5-year-old male mice (n⩾4 per group). Curves are shown to the left. Integrated AUCs (area under curve) are shown to the right. (b) Osteoporosis was analysed in 2.5-year-old male mice (n=3 per group) by microCT. Values of Hounsfield units (HU) and bone mineral density (BMD) for all the femurs are shown. (c) Wound-healing assay in⩾2-year-old mice (n⩾10 per group). (d) Neuromuscular coordination assay. Young (<6 months) and old (>2 years) mice were subjected to the tightrope assay. (e) Levels of p16Ink4amRNA in livers of young (<6 months) and old (⩾2 years) mice (n⩾3 per group) were analysed by quantitative real-time PCR. Data are relative to the levels in young WT mice. (f) Levels of DNA damage in the liver of old (⩾2 years) mice (n⩾3 per genotype) measured as the percentage of 53BP1-foci-positive nuclei by confocal microscopy. In all graphs except panel (d), values are given as average±s.e.m., and statistical analyses are relative to WT controls and determined by the two-tailed Student'st-test: *P<0.05; **P<0.01; ***P<0.005. For panel (d), statistical significance was calculated using Fisher's exact test:#P<0.1. Figure 2: Improved healthy ageing in Sirt1-tg mice. ( a ) Glucose tolerance test (GTT) in 1.5-year-old male mice ( n ⩾ 4 per group). Curves are shown to the left. Integrated AUCs (area under curve) are shown to the right. ( b ) Osteoporosis was analysed in 2.5-year-old male mice ( n =3 per group) by microCT. Values of Hounsfield units (HU) and bone mineral density (BMD) for all the femurs are shown. ( c ) Wound-healing assay in ⩾ 2-year-old mice ( n ⩾ 10 per group). ( d ) Neuromuscular coordination assay. Young (<6 months) and old (>2 years) mice were subjected to the tightrope assay. ( e ) Levels of p16 Ink4a mRNA in livers of young (<6 months) and old ( ⩾ 2 years) mice ( n ⩾ 3 per group) were analysed by quantitative real-time PCR. Data are relative to the levels in young WT mice. ( f ) Levels of DNA damage in the liver of old ( ⩾ 2 years) mice ( n ⩾ 3 per genotype) measured as the percentage of 53BP1-foci-positive nuclei by confocal microscopy. In all graphs except panel ( d ), values are given as average±s.e.m., and statistical analyses are relative to WT controls and determined by the two-tailed Student's t -test: * P <0.05; ** P <0.01; *** P <0.005. For panel ( d ), statistical significance was calculated using Fisher's exact test: # P <0.1. Full size image Another common feature of ageing is the development of osteoporosis, a process that can be promoted by NF-κB [24] , [25] the activity of which is increased during ageing [26] . In agreement with the reported ability of Sirt1 to inhibit NF-κB [15] , [17] , [21] , we observed that Sirt1-tg mice preserved normal bone density values at old age (2.5 years), whereas WT mice showed a significant decline in bone density at this age ( Fig. 2b ). Additional indicators of fitness at old age were obtained by measuring skin regeneration (wound-healing assay, Fig. 2c ) and neuromuscular coordination (tightrope assay, Fig. 2d ), both of which suggested a better performance by Sirt1-tgA mice (no effect at this level was detected in Sirt1-tgB mice). To evaluate ageing at a molecular level, we measured two well-established markers of ageing, namely, the levels of p16 Ink4a mRNA [27] and the accumulation of nuclear foci of DNA damage proteins [28] , [29] . In the case of p16 Ink4a , its transcript levels in liver increased >15-fold in old WT mice compared with young ones (2 years versus 3 months), whereas this increase was significantly attenuated to ∼ 7-fold in Sirt1-tg animals ( Fig. 2e ). Moreover, the number of cells with 53BP1 DNA damage foci in the liver was reduced in old Sirt1-tg mice compared with WT mice of the same age ( Fig. 2f ). Collectively, the analysis of ageing-associated pathologies (glucose intolerance, osteoporosis, decreased wound healing, impaired neuromuscular coordination) and molecular markers of ageing (p16 Ink4a , DNA damage) support the concept that Sirt1 possesses antiageing activity in mammals. Decreased metabolic syndrome-associated liver cancer After analysing the effect of Sirt1 on health and cancer during ageing, we wanted to further extend the cancer studies to a model relevant for metabolic syndrome, a condition that affects up to one-quarter of the human population after middle age [19] , [20] . The array of diseases comprised by metabolic syndrome can be initiated by a high dietary intake and, in the case of liver, results in fatty liver, which can be followed by cirrhosis and finally cancer [18] , [30] . To model metabolic syndrome-associated cancer, we treated mice with a single injection of a hepatic-specific carcinogen, diethylnitrosamine (DEN), followed by continued exposure to HFD. To decrease inter-individual variation due to the hybrid genetic background, all the following assays were performed in mice that had been backcrossed for eight generations with C57BL6 mice and therefore were >99% C57BL6. Furthermore, it is relevant to note that DEN is a poor carcinogen on its own in mice of a C57BL6 genetic background [31] . In fact, most of our WT mice (6 of 11=55%) were completely free of liver tumours at 11 months after treatment with DEN under standard diet conditions. Importantly, all WT mice treated with DEN and under HFD for 11 months developed multiple tumours (on an average 10 tumours) that were quantified and measured in live mice by microcomputed tomography (microCT) ( Fig. 3a ). Notably, the corresponding Sirt1-tg littermate mice presented a significantly lower incidence and burden of liver tumours ( Fig. 3a ). On necropsy, the differences in tumour number and size between WT and Sirt1-tg livers were dramatic ( Fig. 3b ) and histological analyses confirmed that all tumours, both in WT and tg mice, corresponded to liver carcinomas ( Fig. 3c ). We questioned whether the strong protection observed against DEN/HFD-induced hepatocarcinogenesis was also present in other protocols of chemical carcinogenesis. However, when we induced fibrosarcomas with 3-methyl-cholanthrene (3MC), no differences were observed between WT and Sirt1-tg mice ( Fig. 3d ). This differential cancer protection between hepatocytes and fibroblasts correlates with the effect of Sirt1 on DNA damage in the same cell types (see below). We conclude that moderate upregulation of Sirt1 strongly suppresses metabolic syndrome-associated liver cancer. 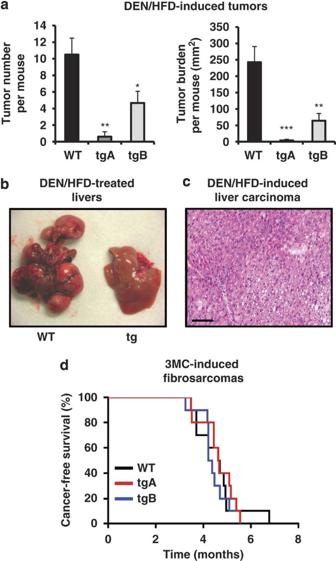Figure 3: Sirt1 protects from metabolic syndrome-associated liver cancer. (a) Tumour number and tumour burden in mice injected with DEN and maintained for 11 months under HFD. Tumours were measured by microCT. Tumour burden per mouse was obtained by adding the areas of the biggest transversal section of each tumour. All assays were performed with male mice (n⩾5 per group). Values are given as average±s.e.m.; statistical analyses are relative to WT controls and determined by the two-tailed Student'st-test: *P<0.05; **P<0.01; ***P<0.005. (b) Macroscopic view of representative livers from littermate mice of the indicated genotypes 11 months after initiation of the DEN/HFD protocol. (c) Histology of a representative liver carcinoma induced by the DEN/HFD protocol. Haematoxylin and eosin staining. The bar indicates 100 μm. (d) Susceptibility to 3MC-induced fibrosarcomas. Mice of the indicated genotypes were injected intramuscularly with 3MC in one of the rear legs and the latency for the development of fibrosarcomas was scored. The log-rank test indicated no significant differences (P>0.6) between genotypes. Figure 3: Sirt1 protects from metabolic syndrome-associated liver cancer. ( a ) Tumour number and tumour burden in mice injected with DEN and maintained for 11 months under HFD. Tumours were measured by microCT. Tumour burden per mouse was obtained by adding the areas of the biggest transversal section of each tumour. All assays were performed with male mice ( n ⩾ 5 per group). Values are given as average±s.e.m. ; statistical analyses are relative to WT controls and determined by the two-tailed Student's t -test: * P <0.05; ** P <0.01; *** P <0.005. ( b ) Macroscopic view of representative livers from littermate mice of the indicated genotypes 11 months after initiation of the DEN/HFD protocol. ( c ) Histology of a representative liver carcinoma induced by the DEN/HFD protocol. Haematoxylin and eosin staining. The bar indicates 100 μm. ( d ) Susceptibility to 3MC-induced fibrosarcomas. Mice of the indicated genotypes were injected intramuscularly with 3MC in one of the rear legs and the latency for the development of fibrosarcomas was scored. The log-rank test indicated no significant differences ( P >0.6) between genotypes. Full size image Hepatic protection from carcinogenic damage Sirt1-tg mice present a lower accumulation of ageing-associated DNA damage in the liver (see above Fig. 2f ), and other investigators have found that Sirt1 contributes to maintain genomic stability [5] , [6] . On the basis of these observations, it can be hypothesized that Sirt1-mediated protection against DEN/HFD-induced liver cancer reflects a dual impact of Sirt1, decreasing the damage produced first by DEN and then by HFD. Although the protection of Sirt1 from HFD-induced damage is well substantiated [15] , [16] , [17] (see also Supplementary Fig. S3 ), nothing is known about the impact of Sirt1 on DEN-induced liver damage. Treatment of mice with DEN under standard feeding conditions triggers a well-known cascade of events in the liver that include DNA damage and apoptosis of centrilobular hepatocytes, production of proinflammatory cytokines and compensatory proliferation [32] . Serum levels of alanine transaminase 48 h after DEN injection already indicated a significant protection from liver injury in Sirt1-tg mice in standard diet ( Fig. 4a ). Immunohistological examination of livers 48 h after DEN showed intense nuclear staining of Sirt1 restricted to the centrilobular regions of the liver (around the central veins) and absent in the periportal regions (around the portal triad) ( Fig. 4b and panoramic views in Supplementary Fig. S5a ). Treatment of in vitro- cultured cells with genotoxic agents recruits Sirt1 to the chromatin [6] , and we questioned whether this also happens in vivo on treating with DEN. Indeed, we observed that DEN increased the amount of chromatin-bound Sirt1 in liver extracts, without detectably affecting the total amount of Sirt1 ( Fig. 4c ). After observing that Sirt1 actively responds to DEN by concentrating in the nucleus and stably binding to chromatin, we examined the impact of Sirt1-tg on the liver on treatment with DEN under standard feeding conditions. Livers from WT mice showed a strong DNA damage response in centrilobular regions, accompanied by high levels of apoptosis and compensatory proliferation ( Fig. 4d and panoramic views in Supplementary Fig. S5b ). Importantly, and in sharp contrast, DEN-treated Sirt1-tg livers showed significantly lower levels of damage, apoptosis and compensatory proliferation ( Fig. 4d and panoramic views in Supplementary Fig. S5b ). DEN is known to require bioactivation by cytochrome CYP2E1 [33] , and we asked whether Sirt1 could be exerting its protective effect by directly affecting DEN metabolism. To address this question, we measured CYP2E1 mRNA levels in control or DEN-treated livers. DEN treatment decreased CYP2E1 levels as previously reported [34] , but no differences in its levels could be observed between WT and Sirt1-tg mice, thus suggesting that Sirt1 does not affect DEN bioactivation ( Fig. 4e ). Next, we wondered whether Sirt1 protection against DNA damage was also detectable in fibroblasts; however, detailed kinetic analyses of γH2AX in individual cells upon treatment with neocarzinostatin could not detect a better repair in Sirt1-tg compared with WT fibroblasts ( Supplementary Fig. S6 ). Our assays suggest a cell-type specificity in the effects of Sirt1 on DNA damage, being more protective in hepatocytes than in fibroblasts. However, the assays and DNA damage agents used here preclude a direct comparison and this point remains to be clarified in future studies. Therefore, overexpression of Sirt1 at the levels achieved in our mouse lines (threefold) significantly protects hepatocytes, but not fibroblasts, from DNA damage, and this correlates with a strong protection against DEN/HFD-induced liver carcinoma but not against 3MC-induced fibrosarcomas (see above, and Fig. 3 ). 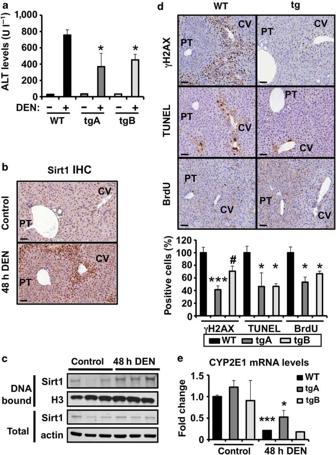Figure 4: Sirt1 protects against DNA damage in the liver. (a) ALT levels in serum before or 48 h after DEN injection (n⩾3 per group). (b) Liver sections stained for Sirt1 before or 48 h after DEN injection in WT mice. The bar indicates 50 μm. (c) Liver protein levels of Sirt1 bound to chromatin or in total extracts from WT mice (n=3) before or 48 h after DEN injection. Histone H3 and actin were used as loading controls. (d) Representative stainings of DNA damage (γH2AX), apoptosis (TUNEL) and compensatory proliferation (BrdU), each showing a centrilobular area (around a centrilobular vein marked as CV) and a portal area (around a portal triad marked as PT) of livers of mice 48 h after DEN injection. Bars indicate 50 μm. Quantifications are shown below relative to WT DEN-treated livers. For quantifications, at least five microscope fields at ×20 magnification, always containing a CV and a PT were scored (n⩾3 per genotype). (e) Levels of CYP2E1 in the livers of control or DEN-treated mice (n⩾3 per group). Differences between tg samples and WT control were not significant (P>0.1) in all cases. In all graphs, values are given as average ± s.e.m., statistical analyses are relative to WT controls and determined by the two-tailed Student'st-test:#P<0.1; *P<0.05; ***P<0.005. Figure 4: Sirt1 protects against DNA damage in the liver. ( a ) ALT levels in serum before or 48 h after DEN injection ( n ⩾ 3 per group). ( b ) Liver sections stained for Sirt1 before or 48 h after DEN injection in WT mice. The bar indicates 50 μm. ( c ) Liver protein levels of Sirt1 bound to chromatin or in total extracts from WT mice ( n =3) before or 48 h after DEN injection. Histone H3 and actin were used as loading controls. ( d ) Representative stainings of DNA damage (γH2AX), apoptosis (TUNEL) and compensatory proliferation (BrdU), each showing a centrilobular area (around a centrilobular vein marked as CV) and a portal area (around a portal triad marked as PT) of livers of mice 48 h after DEN injection. Bars indicate 50 μm. Quantifications are shown below relative to WT DEN-treated livers. For quantifications, at least five microscope fields at ×20 magnification, always containing a CV and a PT were scored ( n ⩾ 3 per genotype). ( e ) Levels of CYP2E1 in the livers of control or DEN-treated mice ( n ⩾ 3 per group). Differences between tg samples and WT control were not significant ( P >0.1) in all cases. In all graphs, values are given as average ± s.e.m., statistical analyses are relative to WT controls and determined by the two-tailed Student's t -test: # P <0.1; * P <0.05; *** P <0.005. Full size image In this study, we provide direct genetic evidence for the antiageing activity of Sirt1 in mammals. We have found that moderate upregulation of Sirt1 expression (threefold) improves healthy ageing but not longevity. Importantly, old Sirt1-tg mice are partially protected from the development of pathologies typically associated with ageing, such as glucose intolerance, osteoporosis and poor wound healing. This improved maintenance of physiological fitness at old ages is accompanied by a decreased expression of molecular markers of ageing in liver, particularly p16 Ink4a mRNA levels and nuclear foci of DNA damage proteins. However, the overall impact on ageing under standard ad libitum feeding conditions was not sufficiently potent to extend longevity. Given the beneficial impact of Sirt1 on ageing, it is tempting to speculate that attaining levels of Sirt1 activity higher than those achieved by us, either genetically or through the use of pharmacological activators, could lead to an extension of the lifespan. Moreover, considering that there are seven different sirtuins in mammalian organisms, it is also possible that several sirtuins must be targeted concurrently to produce lifespan extension. An important observation derived from the analyses of old moribund Sirt1-tg mice is that they are partially protected against spontaneous carcinomas and sarcomas, but not from lymphomas. Other investigators have reported that Sirt1 protects against lymphomas in p53-heterozygous mice [5] , [6] . It is conceivable that Sirt1 has a stronger protective effect against lymphomas with a high degree of genetic instability, such as those developed in p53-heterozygous mice, whereas, spontaneous lymphomas develop less aggressively late in life and are presumably less dependent on protection from acute DNA damage. In the case of spontaneous carcinomas, it is possible that Sirt1 could exert its protective effect through deacetylation and inhibition of β-catenin [7] , which is an oncogene generally associated with epithelial cancers [35] . Together, these factors could explain, at least in part, the differential effect of Sirt1 on ageing-associated carcinomas and sarcomas, versus lymphomas. Caloric restriction (CR) is a well-known manipulation with the ability to delay ageing and increase lifespan [36] . It has been proposed that the beneficial effects of CR in mice are mediated, at least in part, through Sirt1 [37] , [38] , [39] . In this regard, it is interesting to note that our Sirt1-tg mice present an improved glucose tolerance at old age, which is a characteristic feature of CR-treated mice [40] . Further studies are necessary to address the similarities between Sirt1-tg mice under ad libitum conditions and CR-treated mice. In this context, it is also worth to point out the similarities between the phenotypes of our Sirt-tg mice and the reported effects of the small natural compound resveratrol on mice, which upregulates Sirt1 activity, perhaps indirectly through effects mediated by AMPK [13] , [14] . Mice chronically fed with resveratrol are protected from metabolic syndrome induced by HFD [13] , [41] and present improved healthy ageing without affecting longevity [42] . Interestingly, although resveratrol did not protect from spontaneous cancers [42] , our Sirt1-tg mice were partially protected from these cancers. The role of Sirt1 in protection against metabolic syndrome is solidly established [15] , [16] , [17] . On this basis, we have developed a novel carcinogenic protocol to model metabolic syndrome-associated cancer. Metabolic syndrome leads over time to liver steatosis, followed by cirrhosis, which, in turn, is the main risk factor for the development of liver carcinoma [18] , [30] . Specifically, this new experimental cancer model consists of a single injection of the hepatic-specific carcinogen DEN, followed by continued exposure to HFD. This protocol produced a 100% incidence of liver carcinomas in WT C57BL6 mice. Importantly, Sirt1-tg littermate mice were dramatically protected. We show here that the resistance to liver cancer in Sirt1-tg mice is due to a dual protective effect both from the initial acute damage elicited by the carcinogen (DEN) and from the chronic damage produced by HFD. In agreement with previous reports implicating Sirt1 in the maintenance of genomic stability [5] , [6] , we demonstrate here that Sirt1-tg mice are protected from DEN-triggered DNA damage in hepatocytes in vivo . These results reinforce the association between metabolic syndrome and liver cancer, and demonstrate the critical role of Sirt1 in protection from these pathologies. In this context, it is of relevance to mention that recent analyses of Sirt1 expression in various human cancers have found decreased Sirt1 expression in liver cancer, but not in most other human malignancies [5] . Together, our observations demonstrate that chronic and systemic upregulation of Sirt1 is beneficial for health and cancer. Note added in proof : A similar liver cancer mouse model initiated by DEN and promoted by HFD has been reported while this work was under consideration (Park, E.J., Lee, J.H., Yu, G.-Y., He, G., Ali, S.R., Holzer, R.G., Osterreicher, C.H., Takahashi, H. & Karin, M. Cell 140 , 197–208 (2010)). Animal experimentation The Sirt1-tgB line was generated following the same protocol as described for the generation of the Sirt1-tgA line [15] . Both bacterial artificial chromosomes (BAC) were obtained from CHORI (identification numbers: RP23-119G23 for tgA line and RP24-306L15 for tgB line) and purified using the Large-Construct kit (Quiagen). For transgenesis, Sirt1-containing bacterial artificial chromosomes were digested with the restriction enzyme PI- Sce I, thus linearizing them in the vector at a position adjacent to the T7 end of the genomic inserts. Pronuclei of fertilized oocytes, derived from intercrosses between (C57BL6×CBA)F1 mice, were injected with ∼ 2 pl of a DNA solution ( ∼ 1 ng ml −1 ) containing linearized bacterial artificial chromosomes. The resulting offspring was analysed for the presence of transgenes using PCR reactions that amplify sequences from each BAC vector (primers tgA-F 5′-AGATAGTTCACCGGGGTGAGAA-3′; tgA-R 5′-TTCGGTCGAAGAGTATCTGGTG-3′; tgB-F 5′-ACTCTTTAACCGGCCCTTACAAG-3′; tgB-R 5′-TCCTGTGGATCTACCCACTAGTCA-3′). All mice were housed at the serum pathogen-free barrier area of the Spanish National Cancer Research Center (CNIO), Madrid. Mice were treated in accordance with Spanish Laws and the Guidelines for Human Endpoints for Animals Used in Biomedical Research. Mice were observed on a daily basis and killed when they showed signs of morbidity or overt tumours. The genetic background of the mice used in the ageing assays was 87.5% C57BL6 and 12.5% CBA (after two backcrosses). For the rest of the experiments, >99% C57BL6 (after eight backcrosses) mice were used. Mice were fed either with a standard chow diet (Teklad 2018) or with HFD (Research Diets 12451, 45% kJ from fat) when indicated. For the glucose tolerance test, WT and tg mice on both diets were subjected to 6 h of fasting and injected intraperitoneally (i.p.) with 2 g kg −1 glucose, and glucose levels in serum were determined using Glucocard strips (A. Menarini Diagnostics). For the wound-healing assay, wounds were made in the back skin using 4 mm biopsy punches, and healing was measured after 48 h by two researchers blind to the experiment, with the following semiquantitative scoring: 0 for well healed, dry and almost closed wounds; 2 for moist and overtly opened wounds; and 1 for intermediate ones. Osteoporosis was assessed in femurs of live mice on a microCT system (eXplore Vista PET/CT, GE Healthcare), analysing the values obtained from scans acquired with 150 mAmp, 45 kV, 360 projections, 8 shots and 200 μm of resolution. Bone mineral density and Hounsfield unit measurements were obtained using Microwave Software ABA (Advanced Bone Analysis), selecting an area of interest from the femur. For the neuromuscular coordination assay (tightrope), mice were placed on a bar of circular section (60 cm long and 1.5 cm diameter) and the test was considered successful when a mouse stayed on the bar for a cumulative time of at least 60 s throughout five consecutive trials. For the short time response to DEN, 100 mg kg −1 DEN (Sigma) was injected i.p. to <4-month-old males. To determine proliferation, 100 mg kg −1 BrdU (5-bromodeoxyuridine, Sigma) was injected i.p. 2 h before sacrificing the mice. Alanine transaminase levels in serum were determined using VetScan Comprehensive Diagnostic Profile rotors (Abaxis). Mouse tumour models For the DEN/HFD-tumorigenesis model, 16-day-old male mice were injected with 5 mg kg −1 DEN, and then fed on HFD (see above) since weaning. Tumour detection and measurement were performed by microCT in living mice as described for the osteoporosis measurements, except that, in this case, mice were intravenously injected with the iodinated contrast agent Iopamiro 300 (Bracco). Tumour sizes were measured by their largest transversal areas using eXplore Vista software. For the 3MC-tumorigenesis model, 2- to 4-month-old animals were injected intramuscularly in one of the rear legs with 1 mg of 3MC (Sigma) dissolved in 100 μl of corn oil. Mice were observed on a daily basis and killed when the tumours reached a diameter >1.5 cm. Quantitative RT–PCR Total RNA from all tissues was extracted with Trizol (Invitrogen). Reverse transcription was performed using random priming and Superscript Reverse Transcriptase (Life Technologies). Quantitative real-time PCR was performed using DNA Master SYBR Green I mix (Applied Biosystems) in an ABI PRISM 7700 thermocycler (Applied Biosystems). Variations in input RNA were corrected by subtracting the number of PCR cycles obtained for β-actin. Primer sequences are described in Supplementary Table S1 . Protein analyses For isolation of hepatocytes, livers were collected and sliced into small pieces with surgical blades and then incubated at 37 °C for 30 min with 2 mg ml −1 of collagenase (Stem Cell Technologies) solution containing 10 mM HEPES, 136 mM NaCl, 5 mM KCl, 0.5% glucose, 0.7 mM CaCl 2 , 1 mM of dithiothreitol and a cocktail of protease inhibitors. Hepatocytes were then filtered through a 70 μm cell strainer (BD). To isolate chromatin, hepatocytes were resuspended in 200 μl of buffer containing 10 mM HEPES, 10 mM KCl, 1.5 mM MgCl 2 , 0.34 M sucrose and 10% glycerol. Thereafter, Triton X-100 was added to a final concentration of 0.1%. Intact nuclei were spun down and resuspended in a buffer containing 3 mM EDTA and 0.2 mM EGTA, followed by incubation on ice for 30 min. The pellet obtained after spinning down these samples contained the isolated chromatin, which was resuspended in 1× Laemmli buffer. The following antibodies were used: anti-Sirt1 (ab12193, Abcam, 1:2,000), anti-actin (AC-15, Sigma, 1:5,000) and anti-H3 (ab1791, Abcam, 1:1,000), anti-Ac(K310)-p65 (ab19870, Abcam, 1:200) and anti-p65 (sc-8008, Santa Cruz, 1:200). Histological and immunohistochemical methods A detailed histopathological analysis of aged moribund mice was performed by one of the authors (Cañamero, a trained pathologist). Liver sections from DEN-treated mice were stained with the following antibodies: anti-Sirt1 (S5196, Sigma, 1:3,000), anti-BrdU (BU-1, GE Healthcare, 1:100) or anti-γH2AX (JBW301, Millipore, 1:2,000). For TdT-mediated dUTP nick end labelling (TUNEL) stainings, an ApopTag Peroxidase In Situ Apoptosis Detection Kit was used (Millipore). DNA damage in aged livers was assessed by confocal immunofluorescence against 53BP1 (NB100-304, Novus Biologicals, 1:500) on paraffin-embedded sections. For quantifications of DNA damage (γH2AX), apoptosis (TUNEL) and compensatory proliferation (BrdU) in DEN-treated livers, at least five microscope fields at ×20 magnification, and always containing a centrilobular vein and a portal triad, were scored for positive cells ( n ⩾ 3 per genotype). In all graphs, the values represented are relative to WT controls. Statistical analyses Kaplan–Meier curves were compared using the log-rank test. Cancer incidences were compared using Fisher's exact test. All other measurements were compared using the two-tailed Student's t -test. How to cite this article: Herranz, D. et al . Sirt1 improves healthy ageing and protects from metabolic syndrome-associated cancer. Nat. Commun. 1:3 doi: 10.1038/ncomms1001 (2010).